Bio-inspired lanthanum-ortho-quinone catalysis for aerobic alcohol oxidation: semi-quinone anionic radical as redox ligand Oxidation reactions are fundamental transformations in organic synthesis and chemical industry. With oxygen or air as terminal oxidant, aerobic oxidation catalysis provides the most sustainable and economic oxidation processes. Most aerobic oxidation catalysis employs redox metal as its active center. While nature provides non-redox metal strategy as in pyrroloquinoline quinone (PQQ)-dependent methanol dehydrogenases (MDH), such an effective chemical version is unknown. Inspired by the recently discovered rare earth metal-dependent enzyme Ln-MDH, here we show that an open-shell semi-quinone anionic radical species in complexing with lanthanum could serve as a very efficient aerobic oxidation catalyst under ambient conditions. In this catalyst, the lanthanum(III) ion serves only as a Lewis acid promoter and the redox process occurs exclusively on the semiquinone ligand. The catalysis is initiated by 1e - -reduction of lanthanum-activated ortho -quinone to a semiquinone-lanthanum complex La(SQ -. ) 2 , which undergoes a coupled O-H/C-H (PCHT: proton coupled hydride transfer) dehydrogenation for aerobic oxidation of alcohols with up to 330 h −1 TOF. Rare-earth metals are in fact not rare but widely distributed in earth crust and lanthanides such as La and Ce are as abundant as Cu and Zn [1] . In the living sphere, nature has evolved effective strategies in utilizing earth crust metals as active centers in enzymes. However, a rare earth-metal dependent enzyme was not discovered till 2011, when the first lanthanide enzyme, Ln-MDH was discovered in methylotrophic bacterial by Kawai [2] , [3] . Ln-MDH is a lanthanide-dependent methanol dehydrogenase (MDH) [4] , [5] , [6] , closely resembling its calcium counterpart first discovered in 1967 [7] , [8] , [9] . Both MDHs contains a redox-active cofactor, pyrroloquinoline quinone (PQQ) where the oxidation reaction takes place. Mechanistically, the redox cycle between PQQ and its natural substrate methanol proceeds through either an addition-elimination process with a hemiacetal intermediate or direct hydride transfer (Fig. 1a ). In both cases, the active sites metals are believed to serve as only non-redox Lewis acid promoter [10] , [11] , [12] , [13] , [14] , [15] . This mechanistic scenario of Ln-MDH is distinctive from the established alcohol oxidation catalysts wherein redox-active metals such as Pd [16] , [17] , [18] , [19] , [20] , Cu [21] , [22] , [23] , [24] , [25] , [26] , [27] , [28] , and Fe [29] , [30] , [31] , [32] are involved. Fig. 1: Aerobic oxidation of alcohols. a Left: active sites of XoxF-methanol dehydrogenase (La-MDH) (PDB ID: 6adm). Right: overview of methanol dehydrogenase. b Bio-inspired ortho -quinone catalysis. Upper: previous reports about redox properties of PQQ model compounds. Lower: overview of this work. Full size image The unique mechanistic feature of MDH has drawn significant efforts in pursuing bio-inspired catalysis. Ohshiro demonstrated the synthetic application of PQQ in the oxidation of glucose [33] , [34] , [35] , [36] , [37] . Fukuzumi reported a model study of PQQ ester-Ca(ClO 4 ) 2 in the aerobic oxidation of alcohols [10] , [11] . Schelter synthesized a La-MDH model complex and investigated its catalytic performance in the dehydrogenation of benzyl alcohol with ferricenium ion as an oxidant [38] . In the latter two cases, efficient catalytic turnover was only observed in the presence of strong organic base (Note: During the revision of this article, a PQQ biomimetic work ( Chem. Eur. J . 27, 10087-10098 (2021)) demonstrated the oxidation of 4-methyl benzylalcohol still proceeded without DBU, albeit with lower yield), but the efficiency was still too low to be of any synthetic utility, particularly when comparing with the redox-metal catalysts such as Pd [16] , [17] , [18] , [19] , [20] or Cu-nitroxyl [21] , [22] , [23] , [24] , [25] , [26] , [27] , [28] catalytic system in aerobic oxidation. To achieve effective quinone catalysis remains an open challenge from the synthetic point of view, in spite of the ubiquitous existence of quinone-enzyme in nature. Recently, we and others have developed bio-inspired ortho -quinone catalysts with the cofactor of copper amine oxidase, TPQ [39] as a blueprint for the oxidation of amines [40] , [41] , [42] , [43] , [44] , [45] , [46] , [47] , [48] , [49] , [50] , [51] , [52] , [53] , [54] , [55] , [56] , [57] , [58] , [59] , [60] , [61] , [62] . In this work, we report an ortho -quinone/lanthanum complex as highly effective aerobic oxidation catalyst. An open-shell semiquinone anionic radical species in complexing with lanthanum(III) ion is found to serve as the catalytically active species for the oxidation of alcohols under aerobic conditions. The catalysis is initialized by 1e - -reduction of lanthanum-activated ortho -quinone o -Q to a semiquinone-lanthanum complex La( o -Q - . ) 2 , which undergo a concerted dehydrogenation for aerobic oxidation of alcohols with up to 330 h −1 TOF (Fig. 1b ). Establishment of optimal condition We initially found that a three-component system composed of La(OTf) 3 , ortho -quinone o -Q (for the performance of other quinones, see Supplementary Fig. 1 ) and n -Bu 4 NI was active for the aerobic oxidation of benzyl alcohol 1a (Fig. 2a ). A survey of different metal salts indicated all rare earth metals (REE) worked well in the reactions with lanthanum(III) ion as the optimal choice in terms of yields (Fig. 2c ). In contrast, other metals including base metals such as Mg 2+ , Li + , Ca 2+ or redox metals such as Cu 2+ , Fe 3+ or Pd 2+ showed rather poor activity or were even inert (Fig. 2c ). We quickly identified LaI 3 as the optimal choice in lieu of La(OTf) 3 and iodide additive and the two-component catalyst LaI 3 / o -Q was even more active. The reaction reached to completion in 20 mins with only 1 mol% loading of LaI 3 -( o -Q ) 2 (standard condition) (Fig. 2b ), showing significantly improved activity over the best Cu/nitroxyl system (CuOTf/ABNO) [25] . The optimal ratio of La/ o -Q was determined to be 1:2 and further increasing the loading of quinone did not lead to any further improvement (Fig. 2b ). Fig. 2: Selected reaction details. a Control experiment. b Kinetic profile of the reaction. CuOTf/ABNO condition: benzyl alcohol 1a (0.4 mmol), Cu(MeCN)OTf (2 mol %), 4-MeO bpy (2 mol %), ABNO (0.4 mol %), NMI (4 mol %), MeCN (4 mL), room temperature, O 2 balloon. 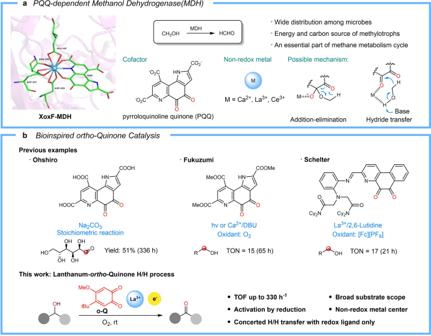Fig. 1: Aerobic oxidation of alcohols. aLeft: active sites of XoxF-methanol dehydrogenase (La-MDH) (PDB ID: 6adm). Right: overview of methanol dehydrogenase.bBio-inspiredortho-quinone catalysis. Upper: previous reports about redox properties of PQQ model compounds. Lower: overview of this work. c Metal screening (for details, see Supplementary Table 1 ). Unless noted, reactions were conducted on a 0.4 mmol scale with 0.6 mL MeCN at room temperature under 1 atm O 2 , and yields were determined by GC using 1,3,5-trimethoxybenzene as internal standard. TBAI = Tetrabutylammonium iodide. ABNO = 9-Azabicyclo[3.3.1]nonane N-oxyl. Full size image Scopes The substrate scope was then explored under the optimal reaction conditions. The reactions worked well with para -substituted benzyl alcohols bearing either electron-donating (Figs. 3 , 2a , b , i ) or electron-withdrawing substituents ( 2c ). The reaction also tolerated functional groups such as thioether ( 2e ), amine ( 2 f ), boronic acid ester ( 2 g ), and free phenols ( 2d and 2 h ), to note that free phenols didn’t work well in the Cu/TEMPO catalysis system [24] . Heterocyclic aromatic alcohols such as ferrocene methanol ( 2 m ) and furfuryl alcohol ( 2n ) and allylic alcohols ( 2j-l ) could be equally applied in the current catalysis. Fig. 3: Substrate scope. Unless otherwise noted, reactions were conducted on a 1 mmol scale with 1 mL MeCN (for aldehyde, lactone and ketone) or MeOH (for ester) at room temperature under 1 atm O 2 , and yields were determined by flash column chromatography. Yields in parentheses were determined by 1 H NMR. For late stage oxidation, reactions were conducted on 0.2 mmol scale with LaI 3 (5 mol%), o -Q (10 mol%) at room temperature under 1 atm O 2 and yields were determined by flash column chromatography (for details, see Supplementary Information). a LaI 3 (2 mol%), o -Q (4 mol%). b LaI 3 (4 mol%), o -Q (8 mol%). c La(OTf) 3 (5 mol%), o -Q (10 mol%), nBu 4 NI (15 mol%) for 2 h. d MeCN/DCM (v/v = 1:1, 0.5 M). Full size image The reactions with aliphatic alcohols have also been examined to give a mixture of aldehyde and ester (from self-condensation). When the reaction was conducted in methanol, a sole formation of methyl ester could be achieved. Selected examples including long-chain alkyl ( 3a and 3b ), cyclopropyl ( 3c ), bulky alkyl ( 3d and 3e ) and piperidinyl ( 3f and 3g ) were listed in Fig. 3 , showing moderate to good activity. Diols such as 1,4-butanediol, 1,5-pentanediol and 1,6-hexanediol could be converted into the corresponding lactones ( 3h-k ) with moderate to high yields. The catalysis also worked extremely well with secondary alcohols including aromatic ( 4aa-af ), allylic alcohols such as verbenol and carveol ( 4c-e ), acyclic ( 4h-i ) and cyclic secondary alcohols ( 4fa-gb ). The alcohols oxidation with testosterone ( 4 m ), androsterone ( 4n ) and estradiol derivates ( 4oa-oc ) went well under this catalysis. Several pharmaceutical intermediates and pesticides were also tested to demonstrate the applicability of our catalysis in the late stage functionalization. Activated benzyl alcohol (Rosuvastatin precursor, 5a ) and primary aliphatic alcohol (Icaridin, 5b ) would be oxidized to corresponding aldehyde and ester with moderate yields. And secondary alcohol (Moxidectin, 5c and Podophyllotoxin, 5d ) proceeded well with nearly quantitative yields. Large scale oxidations were also conducted and more than 200 turnover numbers could be achieved in one hour for benzylic alcohol ( 2a ) and both aromatic and aliphatic alcohols ( 4aa and 4fa ). A competitive one-pot experiment was conducted to investigate the chemoselectivity (Fig. 4a ). It was noted that the reaction rates with secondary alcohol cyclohexanol and those activated primary alcohols such as benzyl alcohol and 1-phenethylalcohol are comparable and they reacted much faster than aliphatic alcohol such as 1-butanol. In comparison, the typical Cu/TEMPO showed significantly preference to primary alcohols over secondary alcohols [24] . Our quinone catalytic system could tolerate free phenol but not free anilines, which is distinctive from Cu-TEMPO system (Fig. 4b ). In oxidizing sluggish 1,6-hexanediol, the quinone catalyst performed slightly better than Cu/ABNO system [26] . Fig. 4: Comparison of our catalyst system with Cu/TEMPO system. a Competition experiments monitored by GC analysis. Standard conditions: LaI 3 (0.004 mmol), o -Q (0.008 mmol), each alcohol substrates (0.1 mmol), MeCN (0.6 mL), room temperature, O 2 balloon. b Comparison of our catalyst system and Cu/TEMPO system. Full size image Control experiments The real active catalytic species was first investigated. In control experiments, removing any of the three catalytic species, o -Q , La(OTf) 3 or TBAI completely shut down the reaction (Fig. 2a ), which implied La 3+ , ortho -quinone catalyst and iodide additive were all essential for this aerobic oxidation. Stoichiometric reactions with either LaI 3 - o -Q or La(OTf) 3 - o -Q -TBAI proceeded smoothly under argon (Fig. 5a , Condition I and II ), suggesting that the substrate-oxidizing active specie was generated from LaI 3 and o -Q , and oxygen served as the terminal oxidant for the recycling of the catalyst. Fig. 5: Control experiment. a Stochiometric reactions. b Other in situ generated semiquinone species control experiments. Yields were based on the amount of La 3+ . c , d Role of iodine. TTF = tetrathiafulvalene. DBU = 1,8-diazabicyclo[5.4.0]undec-7-ene. TBAI 3 = tetrabutylammonium triiodide. Full size image Characterizations and verification of the active species Dramatic color change was noted during the reaction process. When iodide additive was added to a solution of La(OTf) 3 and o -Q , or upon mixing LaI 3 with o -Q , an instant color change from red to dark green was observed (Fig. 6a ) and the color changed back to red when the reaction was complete. UV–visible spectrum of the dark green solution indicated a new absorption at 570 and 750 nm. Previously, similar absorptions were reported for semiquinone radical anion in the presence of metal ion such as Sc(III) or Zn(II) (Fig. 6a ) [63] , [64] . It should be noted a Ce-MDH was crystallized with their active site existed in the form of a Ce(III)-semiquinone anionic radical complex [65] . However, its mechanistic relevance remains obscure. EPR spectrum of the catalytic system confirmed the existence of an organic radical species with g = 2.003 (peak-to-peak linewidth is 1.2 mT) (Fig. 6b ), and the simulation supported a semiquinone radical in coordination with La(III) (Supplementary Fig. 2 ) [66] . In comparison, no obvious EPR signal was detected with only ortho -quinone. Fig. 6: Characterization of active species. a UV–Vis spectrum. Sample concentration: 1.0 mM in MeCN. ( a ): LaI 3 (1.0 mM) and o -Q (2.0 mM); ( b ): La(OTf) 3 (1.0 mM), o -Q (1.0 mM), o -Q red (1.0 mM), DBU (2.0 mM). Inset: The time profile of stoichiometric benzyl alcohol quenching experiment. (Supplementary Fig. 5 ). b EPR spectrum. Sample concentration: LaI 3 (0.1 M) and o -Q (0.2 M) in MeCN at 298 K. c CV test. Sample concentration: 4.0 mM in electrolyte solution (0.1 M nBu 4 NPF 6 in MeCN). d High-resolution mass spectrum of LaI 3 and o -Q in MeCN at 298 K. Full size image Cyclic voltammograms (CV) of o -Q showed a reduction peak at −0.63 V (vs Ag/AgCl), and this was shifted to 0.32 V (vs Ag/AgCl) in the presence of La(OTf) 3 , a positive shift as large as 0.95 V (Fig. 6c ). All the other REE metals also showed large but varied positive shift of the reduction potential of o -Q (Supplementary Fig. 3 ). Hence, the coordination of quinone by coordination to lanthanides [38] could dramatically facilitate its single electron oxidation of iodide (TBAI) ( E ox = 0.39 V vs Ag/AgCl). In comparison, the redox potential gap between free o -Q and TBAI was 1.03 V, largely disfavored for electron transfer [67] , and we did not observe any obvious change when mixing only o -Q and TBAI. Next, reductive initiators other than iodide have been tested and the addition of cobaltocene or tetrathiafulvalene could also initiate the stochiometric reaction with comparable activity (Fig. 5b , Condition III and IV ). Furthermore, the oxidation could also proceed when equal amount of o -Q and hydroquinone o -Q red were employed, such a combination was known to be able to generate semiquinone radical anionic species under basic conditions and this was verified by UV–vis in our case (Fig. 6a and Fig. 5d , Condition V ) [64] . Moreover, adding benzyl alcohol into the dark green solution of LaI 3 /( o -Q ) 2 showed gradually decrease of adsorption as monitored by UV–visible spectroscopy (Fig. 6a ) and increasingly formation of benzaldehyde was observed by GC (Supplementary Fig. 5 ). Similar quenching of the EPR signal was also clearly noted (Fig. 6b ), indicating the consumption of the semiquinone intermediate. Taken together, these results strongly supported the involvement of the reductively generated semiquinone anionic radical in the active catalytic cycle and iodide served as a single electron donor for reductive generation of the active species. We have tried to elucidate the structure of the La(III)-semiquinone complex in both solid and solution phase. Unfortunately, efforts to determine the solid structure by crystalizing the possible complex have been in vain. We then investigated the solution phase complexation between lanthanum (III) and semiquinones by ESI-MS. The MS spectra showed several signals clearly indicating the existence of La-semiquinone complexes (Fig. 6d ). 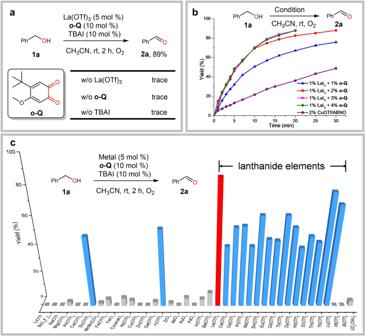Fig. 2: Selected reaction details. aControl experiment.bKinetic profile of the reaction. CuOTf/ABNO condition: benzyl alcohol 1a (0.4 mmol), Cu(MeCN)OTf (2 mol %),4-MeObpy (2 mol %), ABNO (0.4 mol %), NMI (4 mol %), MeCN (4 mL), room temperature, O2balloon.cMetal screening (for details, see Supplementary Table1). Unless noted, reactions were conducted on a 0.4 mmol scale with 0.6 mL MeCN at room temperature under 1 atm O2, and yields were determined by GC using 1,3,5-trimethoxybenzene as internal standard. TBAI = Tetrabutylammonium iodide. ABNO = 9-Azabicyclo[3.3.1]nonane N-oxyl. We were able to identify a major peak at 527.0946, ascribing to the expected 1:2 complex of La( o -Q - . ) 2 + (Fig. 6d ). A minor peak at 721.1922 could also be assigned as La( o -Q - . ) 2 + binding with an additional neutral o - Q , an indication of dynamic and multi- binding behavior between La(III) and quinone/semiquinone. Proposed catalytic cycle Based on the above experimental observations, a catalytic cycle was proposed as shown in Fig. 7a . After coordinating with LaI 3 , o -Q would be reduced by iodide anion via SET to form a radical dianion complex ( Int-1 ) involving a La(III) metal center coordinated with at least two molecules of semiquinone radical anion SQ –∙ . 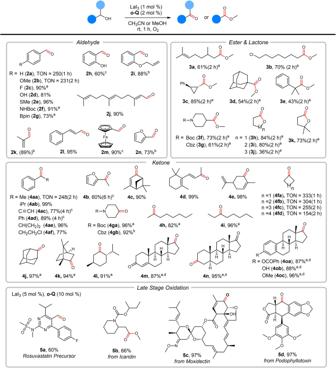Fig. 3: Substrate scope. Unless otherwise noted, reactions were conducted on a 1 mmol scale with 1 mL MeCN (for aldehyde, lactone and ketone) or MeOH (for ester) at room temperature under 1 atm O2, and yields were determined by flash column chromatography. Yields in parentheses were determined by1H NMR. For late stage oxidation, reactions were conducted on 0.2 mmol scale with LaI3(5 mol%),o-Q(10 mol%) at room temperature under 1 atm O2and yields were determined by flash column chromatography (for details, see Supplementary Information).aLaI3(2 mol%),o-Q(4 mol%).bLaI3(4 mol%),o-Q(8 mol%).cLa(OTf)3(5 mol%),o-Q(10 mol%), nBu4NI (15 mol%) for 2 h.dMeCN/DCM (v/v = 1:1, 0.5 M). Alcohol would then coordinate with lanthanum center, following by oxidative dehydrogenation to afford the corresponding aldehyde or ketone. Ester and lactone could be formed via second dehydrogenation from a semi-acetal intermediate. The reduced hydroquinone HQ – complex ( Int-2 ) would be re-oxidized by oxygen to regenerate Int-1 (Fig. 7a ). In the kinetic analysis of the reaction progress, we observed product inhibition effect (Supplementary Fig. 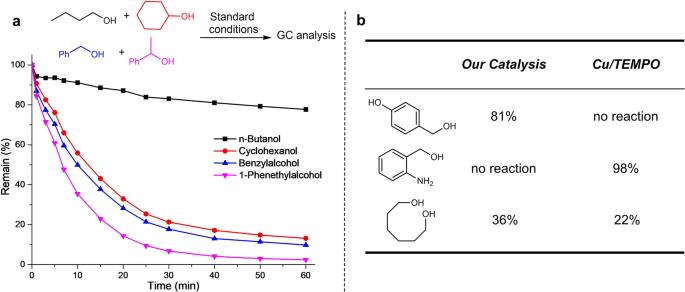Fig. 4: Comparison of our catalyst system with Cu/TEMPO system. aCompetition experiments monitored by GC analysis. Standard conditions: LaI3(0.004 mmol),o-Q(0.008 mmol), each alcohol substrates (0.1 mmol), MeCN (0.6 mL), room temperature, O2balloon.bComparison of our catalyst system and Cu/TEMPO system. 14 ), adding support to the coordination mode. In addition, the preference for ester formation with aliphatic alcohols can also be explained by the relatively strong binding of aliphatic aldehyde with lanthanum metal comparing with benzaldehyde. 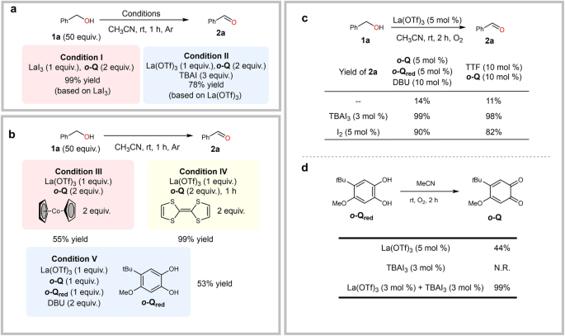Fig. 5: Control experiment. aStochiometric reactions.bOther in situ generated semiquinone species control experiments. Yields were based on the amount of La3+.c,dRole of iodine. TTF = tetrathiafulvalene. DBU = 1,8-diazabicyclo[5.4.0]undec-7-ene. TBAI3= tetrabutylammonium triiodide. Fig. 7: Proposed catalytic cycle and kinetic studies. a Proposed catalytic cycle. b Kinetic isotope effects of benzyl alcohol 1a. c Hammett correlation of para -substituted benzyl alcohols. d Proposed proton-coupled hydride transfer model. Full size image Mechanism of the dehydrogenation process In Fukuzumi and Schelter’s biomimic quinone catalysis, organic base was essential to facilitate the oxidative process and the reactions were believed to proceed via a stepwise deprotonation and hydride transfer mechanism, and the latter step may follow either an addition-elimination or direct hydride transfer pathway. 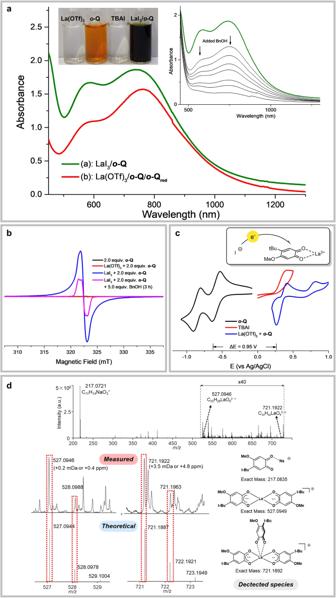Fig. 6: Characterization of active species. aUV–Vis spectrum. Sample concentration: 1.0 mM in MeCN. (a): LaI3(1.0 mM) ando-Q (2.0 mM); (b): La(OTf)3(1.0 mM),o-Q (1.0 mM),o-Qred(1.0 mM), DBU (2.0 mM). Inset: The time profile of stoichiometric benzyl alcohol quenching experiment. (Supplementary Fig.5).bEPR spectrum. Sample concentration: LaI3(0.1 M) ando-Q (0.2 M) in MeCN at 298 K.cCV test. Sample concentration: 4.0 mM in electrolyte solution (0.1 M nBu4NPF6in MeCN).dHigh-resolution mass spectrum of LaI3ando-Q in MeCN at 298 K. 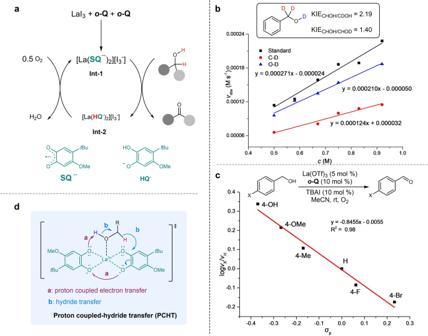Fig. 7: Proposed catalytic cycle and kinetic studies. aProposed catalytic cycle.bKinetic isotope effects of benzyl alcohol 1a.cHammett correlation ofpara-substituted benzyl alcohols.dProposed proton-coupled hydride transfer model. In our case, no obvious base effect was observed (Supplementary Table 6 ) and KIE effect was found on both O–H and C–H of benzylic alcohol (KIE O–H = 1.40, KIE C–H = 2.19) (Fig. 7b ) [68] , [69] , [70] . These observations were supportive of a coupled O–H/C–H hydrogen transfers instead of stepwise deprotonation and hydride transfer. Each of the two semiquinone moieties SQ –∙ may concurrently accept a hydrogen (Fig. 7a ). A Hammett plot with para -substituted benzyl alcohols revealed a preference for electron-rich substitutions with ρ = −0.84 (Fig. 7c ), suggesting that positive charge was developing during H-transfer, an indication of hydride transfer. At this point, the detailed H-transfer mechanism remains to be elucidated, pending further structural characterization of the active intermediate (e.g. Int-1 or Int-2 ). We proposed a proton-coupled hydride transfer (PCHT) pathway to account for the experimental observations (Fig. 7d ). Concerted H-atom transfer, though can not be completely excluded, was unlikely considering the rather low BDE of hydroquinone o -Q red (75 kcal/mol by DFT vs 96 kcal/mol for C-H bond in methanol). The absence of radical-rearrangement products with radical-probe substrates (e.g. 2i , 3c , and 4fa ) also disproved the existence of discrete radical intermediates during hydrogen-transfer, and is in support of hydride transfer. Preliminary DFT calculations were conducted to support the proposed PCHT pathway (Supplementary Fig. 16 ). Inspired by natural lanthanide-dependent enzyme, Ln-MDH, we have developed in this work an efficient LaI 3 / ortho -quinone aerobic oxidation catalyst for alcohol oxidation. The lanthanide- ortho -quinone catalysis demonstrated high activity over a broad range of alcohols, providing practical accesses to aldehydes, ketones as well as esters. Mechanistic studies uncovered that a lanthanum complex with semiquinone radical anion served as the real active catalytic species and the dehydrogenation proceeded most likely via proton coupled-hydride transfer. Though semiquinone radicals are frequently observed in quinoproteins, their function remains obscure. This study implies a possible functioning mode of semiquinone radicals beyond simply positing as a recycling intermediate of quinone cofactors. From the synthetic point of view, the reductive activation strategy as well as the resulted radical anion as redox ligand provides a new twist in exploring aerobic oxidation catalysis. General procedure for alcohol oxidation A flame-dried 10 mL flask was flushed with O 2 and equipped with an O 2 balloon. LaI 3 (5.19 mg, 0.01 mmol) were added to the solution of o -Q (3.88 mg, 0.02 mmol) and alcohol (1.0 mmol) in 1.0 mL of CH 3 CN. The reaction was stirred at room temperature for 1 h. After the reaction was completed, the crude reaction product was purified though a silica gel using 1:10-1:5 EtOAc/petro ether to give a pure product. For some volatile aldehyde, yields were determined by 1 H NMR.